Elucidating heterogeneous photocatalytic superiority of microporous porphyrin organic cage The investigation on the catalytic properties of porous organic cages is still in an initial stage. Herein, the reaction of cyclohexanediamine with 5,15-di[3’,5’-diformyl(1,1’-biphenyl)]porphyrin affords a porphyrin tubular organic cage, PTC-1(2H). Transient absorption spectroscopy in solution reveals much prolonged triplet lifetime of PTC-1(2H) relative to monomer reference, illustrating the unique photophysical behavior of cagelike photosensitizer. The long triplet lifetime ensures high-efficiency singlet oxygen evolution according to homogeneous photo-bleach experiment, electron spin-resonance spectroscopy, and aerobic photo-oxidation of benzylamine. Furthermore, microporous supramolecular framework of PTC-1(2H) is able to promote the heterogeneous photo-oxidation of various primary amines with conversion efficiency above 99% under visible light irradiation. These results indicate the great application potentials of porous organic cages in heterogeneous phase. Visible light photocatalysis provides a green and sustainable approach for the synthesis of valuable organic chemicals by conceptually harnessing solar energy [1] , [2] , [3] , [4] , [5] , [6] , though it is still a great challenge to directly convert visible light to chemical energy because of the lack of absorption in this visible light region for most organic compounds. It has been established that the excited triplet states of some visible light-absorbing molecules are able to initiate the catalytic cycle via photo-induced electron/energy transfer process [1] , [2] , [3] , [4] , [5] , [6] . By virtue of the strong visible light absorption, long triplet lifetime, and high triplet quantum yield, porphyrin derivatives have been extensively utilized as one of the most powerful photocatalysts toward aerobic organic reactions [7] , [8] , [9] , [10] , [11] , [12] , [13] , [14] , [15] , [16] , [17] , [18] . Their practical applications have been retarded by aggregation-induced deactivation of photosensitized performance and low-density solar energy [5] , [15] ; it is therefore of great importance to develop excellent molecular porphyrin photocatalysts with improved absorption and excited states for facilitating photon conversion. Molecular cages such as metal–organic coordination cages and porous organic cages are fabricated from discrete modules mainly depending on coordination and covalent bonds, respectively [19] , [20] , [21] , [22] , [23] , [24] , [25] , [26] , [27] , [28] , [29] , [30] , [31] , [32] , [33] , [34] , [35] , [36] , [37] , [38] , [39] , [40] , [41] , [42] , [43] , [44] , [45] , [46] , [47] , [48] , [49] . These unique synthetic hosts with well-defined cavities are capable of offering diverse weak interactions to recognize and encapsulate organic substrates [46] , constrain their orientations [47] , stabilize intermediates [48] , and mediate reaction kinetics, and thus used for their diverse applications [49] . Although the enzyme-like catalytic activities have been revealed for such special hosts by grafting/post-trapping catalytically active sites on cage skeletons or in cavities, respectively [25] , [44] , [45] , [50] , [51] , [52] , visible light photocatalytic molecular cages toward organic reactions have been still very rarely realized because of the low quantum yield of excited states attributed to the cage-induced self-quenching effect [23] , [53] , [54] , [55] . It has been envisioned that the ultrafast photo-induced energy/electron communication between hosts and cavity-confined guests in a close distance [23] may facilitate the rapid conversion of reaction reagents. In addition, the supramolecular frameworks of molecular cages will possess not only the intrinsic intracage cavities but also the intercage porosities [19] , [27] , [34] , providing a renewable platform for heterogenizing homogeneous photocatalysts. With these considerations in our mind, we plan to develop visible light photocatalytic molecular cages constructed from porphyrin building units for their photo-induced heterogeneous catalysis. In the present work, a [3+6] porous tubular organic cage consisting of three porphyrin units, PTC-1(2H), has been constructed and characterized by single crystal X-ray diffraction analysis. Transient absorption spectroscopy in solution reveals its prolonged triplet lifetime relative to porphyrin monomer, ensuring this kind of porphyrin molecular cage to efficiently promote the visible light-driven evolution of reactive oxygen species (ROS) and thus the aerobic photo-oxidation of benzylamine in homogeneous phase. Furthermore, such prominent molecular photocatalytic activity, in combination with the porous structure of the cage-based supramolecular framework, renders the solid PTC-1(2H) to exhibit 2–5 times faster reaction rate in heterogeneous visible light catalysis of the aerobic photo-oxidation of primary amines than the reference monomer solid and two well-known porphyrin-containing metal‒organic frameworks (MOFs), PCN-222 and PCN-224. These results disclose the great application potential of porous organic cages in visible light heterogeneous photocatalysis. Synthesis of porphyrin organic cage PTC-1(2H) Inspired by the pioneering work of Cooper and co-workers on fabricating the [3+6] porous organic cages including TCC1, TCC2, and TCC3 [56] , a tubular organic cage, PTC-1(2H), composed of porphyrin units was designed through the synthesis pathway (Fig. 1 ). To direct the synthesis, theoretical simulation over the reaction between metal-free 5,15-di[3’,5’-diformyl-(1,1’-biphenyl)]porphyrin (H 2 DBPP) and cyclohexanediamine was carried out, giving a formation energy of −79 kcal mol −1 for the metal-free porphyrin organic cage (Supplementary Data 1 ), consolidating the synthetic feasibility of PTC-1(2H) from thermodynamics by means of such a reaction route; for details, please see Supplementary Information . Subsequent reaction of H 2 DBPP with enantiomerically pure cyclohexanediamine afforded two enantiomers of PTC-1(2H) in a good yield of >85% with the help of trifluoroacetic acid as catalyst. 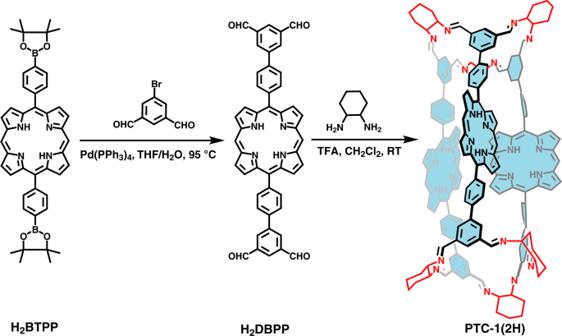Fig. 1: Synthesis of tubular porphyrin organic cage. The synthetic route of PTC-1(2H) includes Suzuki–Miyaura cross-coupling between 5-bromoisophthalaldehyde and 5,15-bis[4-(4,4,5,5-tetramethyl-1,3,2-dioxaborolan-2-yl)phenyl]porphyrin (H2BTPP) together with imine condensation reaction of enantiomerically pure cyclohexanediamine with 5,15-di[3’,5’-diformyl-(1,1’-biphenyl)]porphyrin (H2DBPP). This cage and a monomeric metal-free 5,15-di[3’,5’-cyclohexyliminomethyl-1,1’-biphenyl]porphyrin (H 2 CBPP) were characterized by a series of spectroscopic methods, including nuclear magnetic resonance (NMR), ultraviolet–visible, circular dichroism, and mass spectroscopy (Table 1 and Supplementary Figs. 1 – 12 and Supplementary Table 1 ). Fig. 1: Synthesis of tubular porphyrin organic cage. The synthetic route of PTC-1(2H) includes Suzuki–Miyaura cross-coupling between 5-bromoisophthalaldehyde and 5,15-bis[4-(4,4,5,5-tetramethyl-1,3,2-dioxaborolan-2-yl)phenyl]porphyrin (H 2 BTPP) together with imine condensation reaction of enantiomerically pure cyclohexanediamine with 5,15-di[3’,5’-diformyl-(1,1’-biphenyl)]porphyrin (H 2 DBPP). Full size image Table 1 Photophysical and electrochemical data for H 2 CBPP and PTC-1(2H). Full size table Molecular and supramolecular structures of PTC-1(2H) Purple cubic single crystals of this pair of enantiomers suitable for X-ray diffraction analysis were obtained by diffusing methanol into the chloroform solution of the corresponding compound. The crystal structures of both enantiomers, ( R )-PTC-1(2H) (Fig. 2 ) and ( S )-PTC-1(2H) (Supplementary Fig. 13 ), were determined by X-ray diffraction analysis. 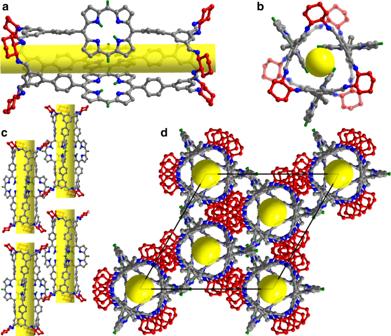Fig. 2: Single crystal structure of molecular organic cage (R)-PTC-1(2H). aSide view andbtop view;cwindow-to-window stacking mode of neighboring molecular organic cages;dpacking profile along the direction of [001] (porphyrin C, gray; cyclohexanediamine C, red; N, blue; H, green; yellow tubes and balls represent the open one-dimensional channel and window, respectively; all selected hydrogen atoms omitted for clarity). Both isostructural enantiomers crystallize in the trigonal system with a chiral R 32 space group (Supplementary Table 2 ), showing six cage molecules per unit cell. Figures 2a and 2b display the molecular structure of ( R )-PTC-1(2H) as representative in side view and top view, respectively. Each cage molecule is composed of 3 porphyrin segments and 6 cyclohexanediimine groups linked by 12 imine bonds, forming a tubular structure with the length of 3.3 nm, which appears to represent one of the longest molecular tube [19] , [20] , [21] , [22] , [23] , [24] , [25] , [26] , [27] , [28] , [29] , [30] , [31] , [32] , [33] , [34] , [35] , [36] , [37] , [38] , [39] , [40] , [41] , [42] , [43] , [44] , [45] , [46] , [47] , [48] , [49] , [50] , [51] , [52] , [53] , [54] , [55] . For each cage molecule, the separation of meso -positional H atom of each porphyrin unit to the N4 mean plane of neighboring porphyrin unit amounts to 2.8510(8) Å, indicating the presence of intramolecular C‒H–π interaction. As shown in the packing diagram for ( R )-PTC-1(2H) (Fig. 2c, d ), the neighboring molecular organic cages are packed into a one-dimensional supramolecular tube depending on Van der Waals force, which are further packed into a three-dimensional porous supramolecular framework depending on Van der Waals interactions as well. In particular, neither intramolecular nor intermolecular neighboring porphyrin units have been arranged in a face-to-face packing mode in the porous cage-based supramolecular framework, enabling the solid sample to exhibit excellent heterogeneous photocatalytic properties through overcoming the general aggregation-induced photocatalyst deactivation for porphyrin materials. It is worth noting that, due to the isostructural nature of PTC-1(2H) enantiomers, subsequent measurements were carried out only on ( R )-PTC-1(2H). Fig. 2: Single crystal structure of molecular organic cage (R)-PTC-1(2H). a Side view and b top view; c window-to-window stacking mode of neighboring molecular organic cages; d packing profile along the direction of [001] (porphyrin C, gray; cyclohexanediamine C, red; N, blue; H, green; yellow tubes and balls represent the open one-dimensional channel and window, respectively; all selected hydrogen atoms omitted for clarity). Full size image Permanent porosity of PTC-1(2H) N 2 sorption experiment at 77 K was conducted to identify the permanent porosity of cage-based framework. PTC-1(2H) shows a typical type I gas sorption behavior with the Brunauer–Emmett–Teller surface area of 112 m 2 g –1 (Fig. 3 ). The large pore size of 1.35 and 2.73 nm for PTC-1(2H) would benefit the small molecule diffusion during catalytic process (Supplementary Fig. 14 ). In addition, the powder X-ray diffraction pattern of the degassed cage-based framework matches well with that of the as-prepared sample, indicating the robust PTC-1(2H) supramolecular framework (Supplementary Fig. 15 ). Fig. 3: N 2 sorption isotherms of PTC-1(2H) at 77 K. Source data are provided as a Source Data file. Full size image Photophysical behaviors of PTC-1(2H) The molecular photophysical behaviors for PTC-1(2H) were studied via electronic absorption, fluorescence, and transient absorption (TA) with monomeric H 2 CBPP as reference. PTC-1(2H) in toluene exhibits a typical electronic absorption spectrum for metal-free porphyrin chromophores with a strong Soret band at 397 nm and four weak Q bands at 506, 542, 580, and 635 nm (Table 1 and Supplementary Fig. 8 ). Only the Soret band of PTC-1(2H) takes a big blue-shift of 15 nm in comparison with that of H 2 CBPP (412 nm) due to the presence of weak intramolecular C‒H–π interaction as revealed in the structure section. In CH 2 Cl 2 and dimethylformamide (DMF), the Soret band and four Q bands of PTC-1(2H) and H 2 CBPP almost do not change (Supplementary Fig. 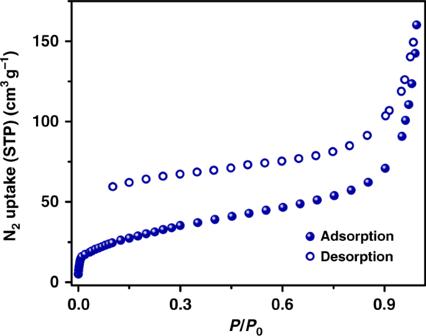Fig. 3: N2sorption isotherms of PTC-1(2H) at 77 K. Source data are provided as a Source Data file. 8 and Supplementary Table 3 ). Upon the excitation at 405 nm, a broad split emission band peaking at 638 and 702 nm was observed for PTC-1(2H) in toluene with an absolute quantum yield of 1.82% and a lifetime of 9.80 ns (Table 1 and Supplementary Figs. 16 – 19 and Supplementary Table 3 ). Both the fluorescence quantum yield and lifetime of PTC-1(2H) are lower than those for H 2 CBPP, namely, 1.86% and 9.87 ns, respectively, due to the presence of much faster non-radiative and intersystem crossing process within the organic cage [57] . Similar phenomenon was also observed in the emission of PTC-1(2H) and H 2 CBPP in CH 2 Cl 2 and DMF, respectively, Supplementary Table 3 . Toward understanding the relaxation process of the organic cage, nanosecond TA spectroscopy under the irradiation of the 355 nm laser pulse was employed. It is worth noting that, before the measurements, the concentration of porphyrin photosensitizers, including PTC-1(2H) and H 2 CBPP reference, was adjusted to keep the same absorption intensity (0.3) at 355 nm. In nitrogen atmosphere, PTC-1(2H) displays the negative absorption band in the range of 370–430 nm due to the typical ground-state bleaching of porphyrin core (Fig. 4a ) [10] , [58] . The positive bands observed at 430–500 nm are attributed to the characteristic porphyrin triplet absorption [10] , [58] . This is also true for the monomeric reference H 2 CBPP with ground-state bleaching and triplet bands observed at 380–425 and 425–500 nm (Supplementary Fig. 20 ). It is worth noting that the triplet quantum yield for either PTC-1(2H) or H 2 CBPP could not be quantitatively evaluated owing to the overlapping between their triplet band and ground-state bleaching band, Fig. 4a and Supplementary Fig. 20a [59] . The similar triplet quantum yield for PTC-1(2H) to that of H 2 CBPP, however, is qualitatively unveiled by their similar absolute fluorescence quantum yield and lifetime [60] , while the triplet lifetime (102.20 μs) for this cage is almost twice longer than that of monomer (53.98 μs), which is associated with the much more rigid structure of the cage molecule (Fig. 4b ) [61] . This result suggests the existence of much more reaction opportunities between the triplet excited states of cages and 3 O 2 molecules, being helpful for the photo-inducing evolution of ROS. The TA spectra of PTC-1(2H) in air are shown (Supplementary Fig. 21 ). Both ground-state bleaching and triplet absorption bands did not show any obvious shift. The triplet lifetime of PTC-1(2H) got seriously shortened to 0.33 μs, in comparison to that in N 2 , 102.20 μs, due to the reaction occurring between the triplet excited states of porphyrin organic cages and O 2 dissolved in solution (Table 1 and Supplementary Fig. 22 ). Fig. 4: Homogeneous photophysical and photocatalytic behaviors of PTC-1(2H). a Nanosecond transient absorption spectra for a toluene solution of PTC-1(2H) excited upon 355 nm laser pulse under nitrogen condition; b normalized kinetic traces of the 450 nm band of PTC-1(2H) and H 2 CBPP under nitrogen condition; c time-dependent absorption spectra of DPBF in DMF upon visible light irradiation ( λ > 510 nm) in the presence of PTC-1(2H); d comparison of absorbance decay rate at 416 nm of DPBF in the presence of different catalysts. Source data are provided as a Source Data file. Full size image Homogeneous photocatalytic property of PTC-1(2H) Prior to evaluating their visible light photocatalytic activity toward ROS evolution, the electrochemical behavior for PTC-1(2H) was studied. Electrochemical measurement result reveals the similar reduction potential of −0.97 V for PTC-1(2H) to −0.98 V for H 2 CBPP due to the very weak intracage interaction as disclosed by theoretically calculated frontier molecular orbitals (Table 1 and Supplementary Figs. 23 and 24 ). The higher reduction potentials of these samples than the reduction potential −0.56 V (vs. standard calomel electrode) for O 2 /O 2 •‒ indicate the photocatalytic capacity of organic cage toward generating O 2 •‒ [62] . This is verified by the subsequent time-dependent photo-bleach experiment based on the oxidation of 1,3-diphenylisobenzofuran (DPBF) by 1 O 2 and O 2 •‒ using PTC-1(2H) as photocatalyst in DMF solution under the visible light irradiation of λ > 510 nm (Fig. 4c and Supplementary Fig. 25 ) [63] . Nevertheless, PTC-1(2H) shows much higher ROS (actually a total 1 O 2 and O 2 •‒ ) generation efficiency than monomeric H 2 CBPP and a typical porphyrin representative of 5,10,15,20-tetraphenylporphyrin (TPP), illustrating the prominent homogeneous photocatalytic property of the cage-like photosensitizer (Fig. 4d ). The higher quantum yield of singlet oxygen for PTC-1(2H) ( Φ Δ = 0.93) than that for H 2 CBPP ( Φ Δ = 0.87) in toluene was quantitatively measured on the basis of the typical emission with the center at ca. 1270 nm with TPP as reference ( Φ Δ = 0.70) [64] (Supplementary Fig. 26 ). This, in cooperation with the similar quantum yield of triplet state for PTC-1(2H) and H 2 CBPP unveiled in a qualitative manner as detailed above, confirms the crucial role of triplet lifetime in the photo-driven singlet oxygen evolution. In addition, the electron spin-resonance (ESR) spectroscopy was also employed to further check the photocatalytic activities of PTC-1(2H) with 2,2,6,6-tetramethylpiperidine (TEMP) and 5,5-dimetyl-1-pyrroline N-oxide (DMPO) as 1 O 2 - and O 2 •‒ -sensitive probes, respectively [63] . The ESR spectra for either TEMP or DMPO trapping agents in the presence of photosensitizer including PTC-1(2H) and three-equivalent H 2 CBPP kept almost silent before the irradiation of a blue light-emitting diode (LED) light (420 nm < λ em < 490 nm) (Supplementary Figs. 27 and 28 ). The irradiation led to an expected appearance of ESR signals for both TEMP and DMPO capturers, indicating the production of 1 O 2 and O 2 •‒ , respectively. In particular, the ESR signal intensity with the 1 O 2 scavenger of TEMP over organic cage is significantly larger than the monomer-induced signal, confirming the outstanding visible light-driven homogeneous photocatalytic properties of PTC-1(2H) in singlet oxygen evolution associated with the long triplet lifetime. In contrast, the similar DMPO-O 2 •‒ ESR signal intensity monitored after addition of organic cage or monomer in a three-equivalent amount indicates their comparable visible light photocatalytic performance in terms of the O 2 •‒ evolution (Supplementary Fig. 28 ). As a total result, the cage triplet lifetime rather than the triplet state quantum yield dominates the present visible light-induced generation of ROS (mainly the singlet oxygen). This result must be helpful in the application of molecular cage in the field of photodynamic therapy and artificial photosynthesis. Further evaluating the photocatalytic properties of PTC-1(2H), the oxidation coupling reaction of benzylamine with 1 O 2 and O 2 •‒ was studied under a blue LED light irradiation. In fact, selective oxidation of amine is of significance in the synthesis of biologically active imine derivatives [65] . With the help of cage-based photocatalyst and within a short time of ca. 15.0 min, >99% benzylamine molecules have been converted into N -benzylidenebenzylamine (based on the NMR data; Table 2 ). In contrast, a longer reaction time of 20.0 and 25.0 min becomes necessary for the monomer photocatalysts, H 2 CBPP and TPP, respectively, to convert >99% benzylamine molecules to target product. This, in cooperation with the TA and ESR spectroscopic results as mentioned above, confirms not only the prominent photocatalytic performance of organic cage under visible light irradiation but also the long triplet lifetime-related promotion mechanism. In the control experiments with reaction exposed in air and in the absence of PTC-1(2H) photocatalyst, the conversion of benzylamine into N -benzylidenebenzylamine either proceeded in much slower speed or kept unreacted, illustrating the crucial role of molecular cage-based photocatalyst and oxygen. Nevertheless, the homogeneous control experiments in the presence of 5.00 μmol triethylenediamine (DABCO) as an efficient singlet oxygen quencher and 5.00 μmol benzoquinone (BQ) as a trapping agent for O 2 •‒ gave 9% and 90% conversion of benzylamine to the corresponding product, respectively (Table 2 ), indicating the more important role of singlet oxygen instead of O 2 •‒ in the present reaction process. Table 2 Homogeneous visible light oxidative coupling of various amines into imines a . Full size table Heterogeneous photocatalytic properties of PTC-1(2H) It is well known that the practical application of the molecular porphyrins as heterogeneous photocatalysts has been retarded by the aggregation-induced deactivation [13] , [15] . The lack of both the intramolecular and intermolecular face-to-face packed porphyrin moieties in the cage-based supramolecular framework as revealed by single crystal X-ray analysis, in combination with the existence of moderately permanent porosity in the PTC-1(2H) framework, therefore inspires our interest toward investigating its heterogeneous photocatalytic performance. For this purpose, the visible light-induced ROS evolution capability of crystalline PTC-1(2H) sample in acetonitrile was examined first. For comparative studies, the ROS evolution activities of solid H 2 CBPP and two well-known porphyrin-containing MOFs of PCN-222 (also known as MOF-545 or MMPF-6) [66] , [67] and PCN-224 [68] were also examined under the same concentration of porphyrin units and experimental conditions. The visible light-induced DPBF photo-bleach time-dependent curves reveal the highest ROS generation efficiency of the solid PTC-1(2H), verifying the expected excellent heterogeneous photocatalytic property of this cage-based supramolecular framework (Fig. 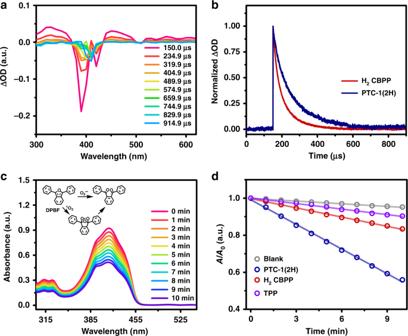Fig. 4: Homogeneous photophysical and photocatalytic behaviors of PTC-1(2H). aNanosecond transient absorption spectra for a toluene solution of PTC-1(2H) excited upon 355 nm laser pulse under nitrogen condition;bnormalized kinetic traces of the 450 nm band of PTC-1(2H) and H2CBPP under nitrogen condition;ctime-dependent absorption spectra of DPBF in DMF upon visible light irradiation (λ> 510 nm) in the presence of PTC-1(2H);dcomparison of absorbance decay rate at 416 nm of DPBF in the presence of different catalysts. Source data are provided as a Source Data file. 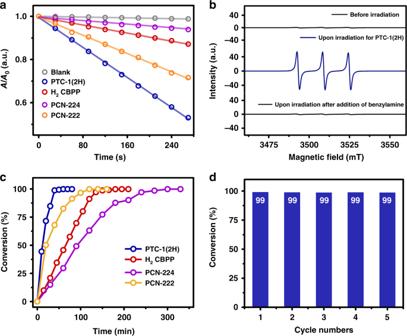Fig. 5: Heterogeneous photocatalytic behavior of PTC-1(2H). aComparison of absorbance decay rate at 410 nm of DPBF in the presence of different photocatalysts in CH3CN upon visible light irradiation ofλ> 510 nm;bESR detection of1O2generation over PTC-1(2H) trapped by TEMP in CH3CN;ccomparison of time-dependent heterogeneous catalytic efficiency of different photocatalysts;drecycle test of PTC-1(2H) in the photo-induced oxidative coupling of benzylamine toN-benzylidenebenzylamine. Source data are provided as a Source Data file. 5a and Supplementary Fig. 29 ). Fig. 5: Heterogeneous photocatalytic behavior of PTC-1(2H). a Comparison of absorbance decay rate at 410 nm of DPBF in the presence of different photocatalysts in CH 3 CN upon visible light irradiation of λ > 510 nm; b ESR detection of 1 O 2 generation over PTC-1(2H) trapped by TEMP in CH 3 CN; c comparison of time-dependent heterogeneous catalytic efficiency of different photocatalysts; d recycle test of PTC-1(2H) in the photo-induced oxidative coupling of benzylamine to N -benzylidenebenzylamine. Source data are provided as a Source Data file. Full size image In addition, visible light-induced photo-oxidation of benzylamine by oxygen was chosen again as a heterogeneous catalytic model reaction. In the oxygen atmosphere, >99% benzylamine in CD 3 CN could be converted into N -benzylidenebenzylamine within only 60 min with the help of PTC-1(2H) supramolecular framework (Table 3 ). ESR spectroscopic data with TEMP and DMPO sensor, respectively, indicate the seriously reduced intensity of photo-induced signals after addition of benzylamine into the suspension of PTC-1(2H) supramolecular framework in CD 3 CN, disclosing the association of high-efficiency conversion of benzylamine with 1 O 2 and O 2 •‒ (Fig. 5b and Supplementary Fig. 30 ) [64] . The heterogeneous control experiments in the presence of the same amount of DABCO and BQ gave 25% and 57% conversion of benzylamine, respectively (Table 3 ), further revealing the more important role of singlet oxygen in the present conversion upon cage photocatalyst. In the control experiments, much longer reaction time of 180, 120, and 300 min were needed for solid H 2 CBPP, PCN-222, and PCN-224, respectively, instead of PTC-1(2H) as heterogeneous photocatalyst to achieve >99% conversion of benzylamine (Fig. 5c and Table 3 ), illustrating the best heterogeneous photocatalytic activity of PTC-1(2H) supramolecular framework among these species. Table 3 Heterogeneous visible light oxidative coupling of various amines into imines a . Full size table After the conversion of benzylamine, the PTC-1(2H) catalyst was separated from the reaction mixture in CD 3 CN and washed by n -hexane for three times to remove the residue chemical over the catalyst surface. 1 H NMR spectroscopic results recorded in CD 3 CN containing dispersed PTC-1(2H) catalyst then clearly reveal the release of N -benzylidenebenzylamine from the pores of the heterogeneous catalyst (Supplementary Fig. 31 ), indicating the effective diffusion of product molecule from the pores within PTC-1(2H) framework due to the big pore size. This might preclude the product inhibition effect [49] and benefit the photo-induced benzylamine conversion. Nevertheless, the highly efficient and constant conversion of benzylamine under the photocatalysis of PTC-1(2H) framework continues for five times, demonstrating the good recyclability of solid PTC-1(2H) catalyst (Fig. 5d ). For the purpose of revealing the general applicability of PTC-1(2H) heterogeneous photocatalyst, the photo-oxidation of a series of primary amine derivatives was carried out. With the assistance of PTC-1(2H) supramolecular framework, the whole series of benzylamine derivatives substituted with different functional groups could be converted to corresponding products with >99% conversion in a specified period, revealing the excellent properties of solid porphyrin organic cage PCT-1(2H) as a heterogeneous photocatalyst (Table 3 ). Among the diverse substrates, (4-fluorophenyl)methanamine converted to N -(4-fluorobenzyl)-1-(4-fluorophenyl)methanimine within the shortest time of 50 min due to the electron-withdrawing effect of fluorine atom. This is also true for 3,4-difluorobenzylamine. In contrast, much longer time ranging from 90 and 120 min becomes necessary for the complete conversion of the chlorine-substituted substrates including 4-chorobenzylamine and 3,4-dichorobenzylamine to corresponding N -benzylidenebenzylamine derivatives due to the effect of the p –π conjugation for chlorine atom [69] . A [3+6] metal-free porphyrin organic cage in a tubular structure with the length of 3.3 nm has been successfully fabricated and assembled into porous supramolecular framework. The cage-induced long triplet lifetime was revealed to play crucial role in the high-efficiency singlet oxygen evolution and in turn the photo-oxidation of benzylamine in homogeneous phase. More importantly, the porphyrin cage-based porous supramolecular framework overcomes the general aggregation-induced deactivation of molecular porphyrins as heterogeneous catalyst and efficiently promotes photo-oxidation coupling reaction of various primary amines. The present result discloses the unique catalytic activity of porous organic cages in heterogeneous photocatalysis associated with the unique cage-induced long triplet lifetime and porous structure, which is expected to ignite more research interest toward exploration of porous organic cage with great heterogeneous application potentials. Remark Dichloromethane was freshly distilled from CaH 2 . The other commercial chemicals were used without any further treatment. H 2 DBPP was prepared from the reaction between 5,15-bis[4-(4,4,5,5-tetramethyl-1,3,2-dioxaborolan-2-yl)phenyl]porphyrin [70] and 5-bromoisophthalaldehyde. For details, please see Supplementary Information . Synthesis of PTC-1(2H) To a suspension of H 2 DBPP (0.06 mmol) and trifluoroacetic acid (2.0 μL) in dichloromethane (50 mL), a solution of enantiomerically pure cyclohexanediamine (14.8 mg, 0.130 mmol) in dichloromethane (20 mL) was added slowly. The mixture was stirred at room temperature for 24 h. Then the reaction mixture was evaporated under reduced pressure and applied on a silica gel column using tetrahydrofuran as eluent. Repeated column chromatography followed by recrystallization in chloroform and methanol gave the target organic cages as dark red powder in the yield of 85.6% and 87.3% for ( R )-PTC-1(2H) and ( S )-PTC-1(2H), respectively. 1 H NMR (400 MHz, CDCl 3 ): δ 8.78 (d, J = 4.5 Hz, 12H), 8.64 (d, J = 16.3 Hz, 12H), 8.54 (s, 6H), 8.37 (d, J = 7.6 Hz, 12H), 8.23 (s, 6H), 8.16 (d, J = 7.7 Hz, 12H), 8.07 (s, 6H), 7.75–7.45 (m, 18H), 3.71 (dd, J = 14.0, 8.8 Hz, 6H), 3.57 (dd, J = 15.4, 8.5 Hz, 6H), 2.00 (d, J = 11.8 Hz, 24H), 1.70 (s, 24H), -3.56 (s, 6H); 13 C NMR (100 MHz, CDCl 3 ): δ 160.67, 160.31, 146.71, 144.34, 141.13, 141.02, 139.18, 137.44, 137.19, 135.18, 132.51, 131.32, 130.04, 125.63, 118.11, 104.50, 75.66, 74.99, 33.27, 32.81, 29.70, 24.68; MS (MALDI-TOF) m / z : [M]+calcd. for C 180 H 150 N 24 , 2649.25; found: 2649.53 for ( R )-PTC-1(2H) and 2649.34 for ( S )-PTC-1(2H); analysis of ( R )-PTC-1(2H) (calcd., found for C 180 H 150 N 24 ·1.5CHCl 3 ): C (77.07, 76.96), H (5.40, 5.88), N (11.89, 11.66); analysis of ( S )-PTC-1(2H) (calcd., found for C 180 H 150 N 24 ): C (81.60, 81.22), H (5.70, 5.44), N (12.69, 12.87).